Macrophages monitor tissue osmolarity and induce inflammatory response through NLRP3 and NLRC4 inflammasome activation Interstitial osmolality is a key homeostatic variable that varies depending on the tissue microenvironment. Mammalian cells have effective mechanisms to cope with osmotic stress by engaging various adaptation responses. Hyperosmolality due to high dietary salt intake has been linked to pathological inflammatory conditions. Little is known about the mechanisms of sensing the hyperosmotic stress by the innate immune system. Here we report that caspase-1 is activated in macrophages under hypertonic conditions. Mice with high dietary salt intake display enhanced induction of Th17 response upon immunization, and this effect is abolished in caspase-1-deficient mice. Our findings identify an unknown function of the inflammasome as a sensor of hyperosmotic stress, which is crucial for the induction of inflammatory Th17 response. Our current understanding of the mechanisms sensing stress within tissue microenvironment is limited. Much attention has been focused at cellular stress responses, where dedicated sensors, such as heat shock transcription factor 1 (HSF-1), hypoxia-inducible factor 1-alpha (HIF-1α) and nuclear factor of activated T cell 5 (NFAT5), detect different stress conditions (that is, heat shock, hypoxia and hyperosmotic stress, respectively) and mediate cell-autonomous adaptations that enable a cell to survive unfavourable environmental conditions [1] , [2] , [3] . However, growing evidence implicates cellular stress responses in a number of chronic inflammatory conditions, such as type-2 diabetes, atherosclerosis, inflammatory bowel diseases and neurodegenerative diseases [4] , [5] , [6] , [7] , [8] , suggesting a potential role of inflammation as the adaptive response to stress conditions. Inflammation is a protective response that enables survival during infection or injury and maintains tissue homeostasis under a variety of noxious conditions [9] . Inflammatory responses are typically initiated by the innate immune system, when cells such as macrophages and mast cells detect noxious stimuli (for example, infection and tissue injury). Some noxious stimuli can be detected based on associated structural features, such as pathogen-associated molecular patterns [10] . This mode of recognition is mediated by pattern-recognition receptors, including Toll-like receptors, C-type lectin receptors, as well as cytosolic Nod-like receptors (NLRs) and retinoic acid-inducible gene 1 (RIG-I)-like helicases [11] . Other noxious challenges cannot be detected based on structural recognition and their detection relies instead on functional features, such as enzymatic activities, membrane pore formation and de-sequestration of cellular components. This second mode of sensing is not well characterized with the exception of NLRP3 inflammasome-mediated detection of noxious stimuli [12] , [13] , [14] . The activation of caspase-1 by inflammasomes is a key signalling pathway for inflammation, which is mediated by certain NLRs, often in response to microbes [15] , [16] . Several distinct NLR-containing inflammasomes have been identified, including NLRP3 and NLRC4. Inflammasomes are molecular platforms that drive the proteolytic activation of caspase-1 and caspase-11, which results in the secretion of mature, biologically active interleukin (IL)-1β and IL-18 (refs 17 , 18 ). Recent studies have shown that various stimuli of either biological or non-biological origin can activate the NLRP3 inflammasome, including ATP [19] , bacterial pore-forming toxins [19] , [20] , alum [21] and several types of crystals [22] , [23] , [24] , [25] , suggesting that NLRs can sense common cellular stress events that are triggered by these diverse stimuli. Consistent with this idea, potassium (K + ) efflux [26] , calcium (Ca 2+ ) influx [27] , lysosomal membrane disruption [24] and mitochondrial reactive oxygen species (ROS) production [28] have been implicated as the key cellular events that induce the assembly and activation of the NLRP3 inflammasome. These cellular events, and in particular the ROS production, are often associated with diverse stress conditions. Together, these observations suggest that NLRP3 inflammasomes function to detect certain stress conditions and to translate them into inflammatory responses. Consistent with this notion, here we identify a previously unknown function of the inflammasome as a sensor of hyperosmotic stress. We show that caspase-1 is activated in macrophages exposed to hypertonic conditions, which in turn triggers the release of mature IL-1β. This caspase-1 activation requires both NLRP3 and NLRC4 inflammasomes and is regulated by autophagy through controlling mitochondrial ROS production. We confirm our observations in vivo , showing that hyperosmotic stress induces caspase-1/NLRP3/NLRC4-dependent peritoneal inflammation. Moreover, mice with high dietary salt (NaCl) intake have higher inflammatory Th17 response upon immunization, which is abolished in caspase-1-deficient mice. Macrophages secrete IL-1β in response to hyperosmotic stress To investigate the potential inflammatory response to hyperosmotic stress by macrophages, addition of NaCl, sorbitol or glucose into the culture medium of cells (that is, osmotic increase) was used to generate hypertonic conditions. Bone marrow-derived macrophages (BMDMs) exposed to these hypertonic conditions, as expected, experienced acute cell shrinkage within the first minute and were able to restore near-normal cell volume by 30 min ( Fig. 1a,b ), demonstrating an induction of adaptation response in order to counteract the initial insult. Early-stress response genes, such as Hsph1 , Ier3 and Gadd45γ , were induced in BMDMs as measured by genome-wide microarray analysis of gene expression ( Fig. 1c ). Moreover, a subset of genes induced by lipopolysaccharide (LPS), including Ccl2 , Ccl7 and Cxcl2 , were also observed in BMDMs following the exposure to the hypertonic conditions (both NaCl and sorbitol; Fig. 1c ), suggesting that inflammatory signalling pathways could be also involved in the non-cell autonomous adaptation response to hyperosmotic stress. We therefore hypothesized that in addition to the cell autonomous adaptation, hyperosmotic stress in macrophages may also lead to an inflammatory response to promote tissue level adaptations. 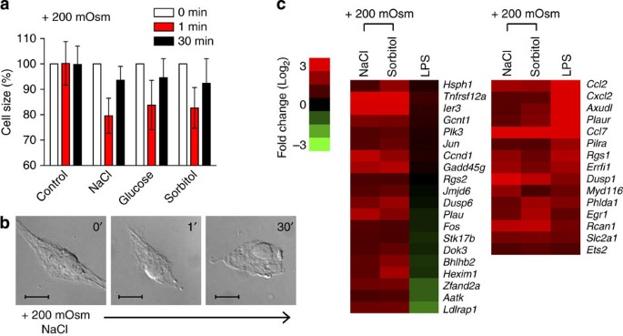Figure 1: Hyperosmotic stress induces adaptation response in macrophages. (a,b) BMDMs were maintained in isotonic conditions (controls) or switched to hypertonic conditions (+200 mOsm) by adding NaCl, glucose or sorbitol. Cell size was measured by using a Coulter counter (a) or observed by microscopy (b) at the indicated times. (c) Heat map displaying microarray data, fold change of selected gene subset in BMDMs incubated in hypertonic conditions (NaCl or sorbitol) or stimulated with LPS for 3 h. Only genes with a significant fold change are presented. Data ina,bare representative of two independent experiments. Data inaare the mean±s.d. of 1 × 103cells counted. Scale bar, 10 μm. Figure 1: Hyperosmotic stress induces adaptation response in macrophages. ( a , b ) BMDMs were maintained in isotonic conditions (controls) or switched to hypertonic conditions (+200 mOsm) by adding NaCl, glucose or sorbitol. Cell size was measured by using a Coulter counter ( a ) or observed by microscopy ( b ) at the indicated times. ( c ) Heat map displaying microarray data, fold change of selected gene subset in BMDMs incubated in hypertonic conditions (NaCl or sorbitol) or stimulated with LPS for 3 h. Only genes with a significant fold change are presented. Data in a , b are representative of two independent experiments. Data in a are the mean±s.d. of 1 × 10 3 cells counted. Scale bar, 10 μm. Full size image To examine whether the inflammasome is activated by hyperosmotic stress, BMDMs were exposed to hypertonic conditions after priming with LPS to allow the expression of pro-IL-1β. There was no IL-1β or IL-6 secretion observed in non-primed BMDMs ( Fig. 2a ). However, after LPS priming, IL-1β secretion was induced in BMDMs incubated in hypertonic conditions with NaCl or glucose, whereas IL-6 secretion was observed in both isotonic and hypertonic conditions ( Fig. 2a ), suggesting that hyperosmotic stress induces the processing and release of mature IL-1β. Notably, the secretion of IL-1β by hypertonic stress was at a lower range as compared with that by the known inflammasome-activating agents such as ATP and alum ( Fig. 2a ). Similar results were also observed in macrophage cell line J774 ( Supplementary Fig. 1 ). Moreover, hyperosmotic stress also induced the release of IL-1α ( Fig. 2a ), which, like IL-1β, has been shown to rely on caspase-1 activity [29] . 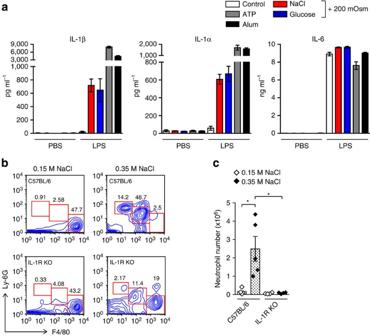Figure 2: Hyperosmotic stress induces IL-1β secretion in macrophages. (a) BMDMs primed without (PBS) or with LPS were incubated overnight in isotonic conditions (control) or hyperosmotic conditions (+200 mOsm) by adding NaCl, glucose or sorbitol, or stimulated with ATP (5 mM) or alum (250 μg ml−1) for 2 or 6 h, respectively. IL-1β, IL-1α and IL-6 in media supernatants were measured by ELISA. (b,c) Wild-type (C57BL/6) or IL-1R-deficient mice (IL-1R KO) were injected peritoneally with 0.15 M (‘isotonic’) or 0.35 M (‘hypertonic’) of NaCl (each group,n=4). Peritoneal lavage cells were analysed for neutrophils after 16 h. Contour plots of fluorescence-activated cell sorting analysis show the percentages of neutrophils (Ly-6G+, F4/80 negative), inflammatory monocytes (Ly-6G+, F4/80+low) and resident macrophages (Ly-6G negative, F4/80+high) cells (b). Neutrophil numbers were determined by using cell-counting beads as described in the Methods (c). Data are representative of three (a,b) independent experiments. Data indicate mean±s.d. of quadruplicates (a), or for pooled groups of mice from three experiments (c). Student’st-test: *P≤0.05. Figure 2: Hyperosmotic stress induces IL-1β secretion in macrophages. ( a ) BMDMs primed without (PBS) or with LPS were incubated overnight in isotonic conditions (control) or hyperosmotic conditions (+200 mOsm) by adding NaCl, glucose or sorbitol, or stimulated with ATP (5 mM) or alum (250 μg ml −1 ) for 2 or 6 h, respectively. IL-1β, IL-1α and IL-6 in media supernatants were measured by ELISA. ( b , c ) Wild-type (C57BL/6) or IL-1R-deficient mice (IL-1R KO) were injected peritoneally with 0.15 M (‘isotonic’) or 0.35 M (‘hypertonic’) of NaCl (each group, n =4). Peritoneal lavage cells were analysed for neutrophils after 16 h. Contour plots of fluorescence-activated cell sorting analysis show the percentages of neutrophils (Ly-6G + , F4/80 negative), inflammatory monocytes (Ly-6G + , F4/80 +low ) and resident macrophages (Ly-6G negative, F4/80 +high ) cells ( b ). Neutrophil numbers were determined by using cell-counting beads as described in the Methods ( c ). Data are representative of three ( a , b ) independent experiments. Data indicate mean±s.d. of quadruplicates ( a ), or for pooled groups of mice from three experiments ( c ). Student’s t -test: * P ≤0.05. Full size image IL-1β has a key function in the recruitment of neutrophils, and the IL-1β-dependent peritoneal accumulation of neutrophils can be used as an in vivo assay for IL-1β production [22] , [25] , [30] . Using this model we found that intraperitoneal (i.p.) injection of hypertonic NaCl (0.35 M) but not isotonic NaCl (0.15 M) induced influx of neutrophils (Ly-6G + , F4/80 − ) and inflammatory monocytes (Ly-6G + , F4/80 +low ) into the peritoneal cavity ( Fig. 2b ). Importantly, neutrophil influx into the peritoneal cavity induced by high NaCl was largely abolished in IL-1 receptor-deficient mice ( Fig. 2b,c ). Together, these observations demonstrate that hypertonic stress can induce IL-1-dependent inflammatory response in vivo. Hyperosmotic stress activates caspase-1 to release IL-1β We next tested whether hyperosmotic stress activates caspase-1, which is necessary for processing and secretion of IL-1β. Immunoblot analysis of cell lysates from BMDMs showed that addition of NaCl, glucose or sorbitol (that is,+200 mOsm) into the culture medium induced the cleavage of caspase-1 into the active subunit p10 ( Fig. 3a ) and its release into the culture medium ( Fig. 3b ). This caspase-1 cleavage was also demonstrated in macrophage cell line J774 but not in other cell types, such as mouse embryonic fibroblasts, L929 cells and Hepa cells ( Supplementary Fig. 3 ), suggesting that hyperosmotic stress-induced activation of caspase-1 is not ubiquitous and may be macrophage specific. Consistently, dose- and time-dependent activation of caspase-1 in BMDMs was observed specifically upon hyperosmotic challenge to BMDMs ( Fig. 3c ). The activation of caspase-1 was also demonstrated by using FLICA, a fluorescent inhibitor that binds covalently to the active caspase-1 ( Fig. 3d ). To confirm that the IL-1β secretion by hyperosmotic stress was caspase-1-dependent, caspase-1-deficient BMDMs were used. Only minimal release of IL-1β was observed as compared with BMDMs from wild-type mice ( Fig. 3e ). We also measured lactate dehydrogenase in the supernatants as an indicator of cell viability, which confirmed that there was no obvious cytotoxicity under hypertonic conditions ( Supplementary Fig. 4 ). Collectively, these results suggest that caspase-1 is activated in the inflammasome complex upon hyperosmotic challenge, leading to the processing and secretion of IL-1β. 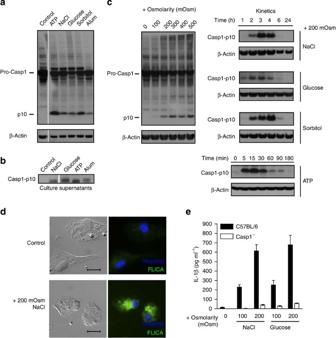Figure 3: Hyperosmotic stress induces caspase-1 activation and caspase-1-dependent IL-1β secretion. (a–d) BMDMs primed with LPS were maintained in isotonic conditions (control) or switched to hyperosmotic conditions (+200 mOsm (a,b) or as indicated (c,d)) by adding NaCl, glucose or sorbitol for 3 h (a,c,d), overnight (b) or for the indicated times (c). LPS-primed BMDMs stimulated with ATP (5 mM) for 30 min (a), 2 h (b) or the indicated times (c), or with alum (250 μg ml−1) for 4 h (a) or 6 h (b), were used as positive controls. The cleavage of caspase-1 to its active p10 subunit in BMDMs was detected by immunoblot analysis in cell lysates (a,c) or in media supernatants (b; see alsoSupplementary Fig. 2a), or the caspase-1 activation was visualized by incubation with a fluorescent cell-permeable probe that binds only to activated caspase-1 (FLICA;d). Scale bar, 10 μm. (e) Wild-type (C57BL/6) or caspase-1-deficient (Casp1−/−) BMDMs primed with LPS were incubated overnight in isotonic conditions (+0 mOsm) or hypertonic conditions (+100 or 200 mOsm). IL-1β in media supernatants was measured by ELISA. Data are representative of three independent experiments. Data ineare the mean±s.d. of quadruplicates. Figure 3: Hyperosmotic stress induces caspase-1 activation and caspase-1-dependent IL-1β secretion. ( a – d ) BMDMs primed with LPS were maintained in isotonic conditions (control) or switched to hyperosmotic conditions (+200 mOsm ( a , b ) or as indicated ( c , d )) by adding NaCl, glucose or sorbitol for 3 h ( a , c , d ), overnight ( b ) or for the indicated times ( c ). LPS-primed BMDMs stimulated with ATP (5 mM) for 30 min ( a ), 2 h ( b ) or the indicated times ( c ), or with alum (250 μg ml −1 ) for 4 h ( a ) or 6 h ( b ), were used as positive controls. The cleavage of caspase-1 to its active p10 subunit in BMDMs was detected by immunoblot analysis in cell lysates ( a , c ) or in media supernatants ( b ; see also Supplementary Fig. 2a ), or the caspase-1 activation was visualized by incubation with a fluorescent cell-permeable probe that binds only to activated caspase-1 (FLICA; d ). Scale bar, 10 μm. ( e ) Wild-type (C57BL/6) or caspase-1-deficient (Casp1 −/− ) BMDMs primed with LPS were incubated overnight in isotonic conditions (+0 mOsm) or hypertonic conditions (+100 or 200 mOsm). IL-1β in media supernatants was measured by ELISA. Data are representative of three independent experiments. Data in e are the mean±s.d. of quadruplicates. Full size image Hyperosmotic stress activates both NLRP3 and NLRC4 inflammasomes To determine which NLR protein is involved in cell response to hypertonic stress, we used BMDMs from mice deficient in NLRP3, the adaptor molecule ASC or NLRC4. Upon hyperosmotic challenge, BMDMs lacking NLRP3, ASC or NLRC4 had minimal or reduced activation of caspase-1 as compared with BMDMs from wild-type animals ( Fig. 4a ), indicating that both NLRP3 and NLRC4 inflammasomes are required for caspase-1 activation. We therefore also tested BMDMs lacking both NLRP3 and NLRC4, and confirmed that further reduction of caspase-1 activation was observed in these cells ( Fig. 4a ). The requirement of both NLRP3 and NLRC4 in caspase-1 activation by hyperosmotic stress was further confirmed by measuring IL-1β secretion, where BMDMs lacking either of NLRP3, ASC or NLRC4 had reduced IL-1β secretion, whereas BMDMs lacking both NLRP3 and NLRC4 had minimal IL-1β secretion, similar to that by caspase-1-deficient BMDMs ( Fig. 4b ). In contrast, BMDMs lacking NLRP3 or NLRC4 produced minimal or normal IL-1β release, respectively, in response to ATP ( Fig. 4b ), the known activator for NLRP3 inflammasome [19] . These results suggest that NLRP3 and NLRC4 inflammasomes are responsible for sensing hyperosmotic stress in macrophages. In line with these findings, mice lacking NLRP3 and NLRC4 recruited significantly fewer neutrophils into the peritoneal cavity than wild-type mice after injection of high NaCl ( Fig. 4c ). 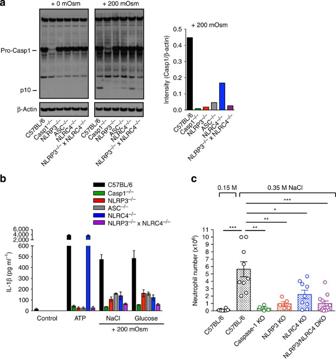Figure 4: Hyperosmotic stress activates NLRP3 and NLRC4 inflammasomes. (a,b) LPS-primed BMDMs generated from wild-type (C57BL/6), Casp1−/−, NLRP3−/−, ASC−/−NLRC4−/−or NLRP3−/−× NLRC4−/−mice were incubated for 3 h (a) or overnight (b) in isotonic conditions (+0 mOsm; control) or hypertonic conditions (+200 mOsm) by adding NaCl (a,b) or glucose (b). The cleavage of caspase-1 to its active p10 subunit in BMDMs was detected by immunoblot analysis in cell lysates (a). IL-1β in supernatants was measured by ELISA (b). (c) Wild-type mice (C57BL/6;n=8) or mice deficient in genes encoding caspase-1 (n=4), NLRP3 (n=5), NLRC4 (n=9) or NLRP3/NLRC4 (double knockout, DKO;n=11) were injected peritoneally with 0.35 M (‘hypertonic’) NaCl, or wild-type mice (C57BL/6;n=8) with 0.15 M (‘isotonic’) NaCl. Peritoneal lavage cells were analysed for neutrophils after 16 h. Data are representative of three independent experiments (a,b). Data indicate mean±s.d. of quadruplicates (b), or mean for pooled groups of mice from two to three experiments (c). Student’st-test: *P≤0.05, **P≤0.01, ***P≤0.001. Figure 4: Hyperosmotic stress activates NLRP3 and NLRC4 inflammasomes. ( a , b ) LPS-primed BMDMs generated from wild-type (C57BL/6), Casp1 −/− , NLRP3 −/− , ASC −/− NLRC4 −/− or NLRP3 −/− × NLRC4 −/− mice were incubated for 3 h ( a ) or overnight ( b ) in isotonic conditions (+0 mOsm; control) or hypertonic conditions (+200 mOsm) by adding NaCl ( a , b ) or glucose ( b ). The cleavage of caspase-1 to its active p10 subunit in BMDMs was detected by immunoblot analysis in cell lysates ( a ). IL-1β in supernatants was measured by ELISA ( b ). ( c ) Wild-type mice (C57BL/6; n =8) or mice deficient in genes encoding caspase-1 ( n =4), NLRP3 ( n =5), NLRC4 ( n =9) or NLRP3/NLRC4 (double knockout, DKO; n =11) were injected peritoneally with 0.35 M (‘hypertonic’) NaCl, or wild-type mice (C57BL/6; n =8) with 0.15 M (‘isotonic’) NaCl. Peritoneal lavage cells were analysed for neutrophils after 16 h. Data are representative of three independent experiments ( a , b ). Data indicate mean±s.d. of quadruplicates ( b ), or mean for pooled groups of mice from two to three experiments ( c ). Student’s t -test: * P ≤0.05, ** P ≤0.01, *** P ≤0.001. Full size image Hyperosmotic stress activates inflammasomes via mitochondrial ROS Although the proximal mechanisms of inflammasome activation are still poorly understood, there are at least three requirements that have been suggested for NLRP3 inflammasome activation: potassium (K + ) efflux, calcium (Ca 2+ ) influx, phagolysosomal membrane rupture and ROS generation [24] , [26] , [27] , [28] . We tested these requirements in our system in order to gain insight into the mechanism involved in hyperosmotic stress-induced inflammasome activation. As expected, inhibition of K + efflux by high extracellular KCl, and inhibition of Ca 2+ influx by extracellular and intracellular Ca 2+ chelators, or blocking phagocytosis by cytochalasin D inhibited inflammasome activation by ATP or alum; however, these treatments did not inhibit caspase-1 activation by hypertonic stress ( Fig. 5a , Supplementary Fig. 5 and Fig. 6a ), presumably because it relies on both NLRP3 and NLRC4. The response was also unaffected in macrophages lacking P2X 7 receptor that could possibly sense endogenous ATP released from cells under hypertonic conditions ( Supplementary Fig. 6b ). In contrast, treatment of macrophages with ROS inhibitor N -acetyl- L -cysteine (NAC) blocked caspase-1 activation by hyperosmotic stress ( Fig. 5a ). NAC also inhibited the secretion of IL-1β ( Fig. 5b ), although this effect is compounded by the effect of NAC on IL-1 gene transcription [31] . To further confirm the ROS dependency, we used another ROS inhibitor ebselen to treat macrophages, and observed similar results ( Fig. 5c ). Furthermore, there was no obvious cytotoxic or off-target effect of the ROS inhibitors ( Supplementary Fig. 7 ). Together, these results indicate that ROS is required for hyperosmotic stress-induced inflammasome activation. 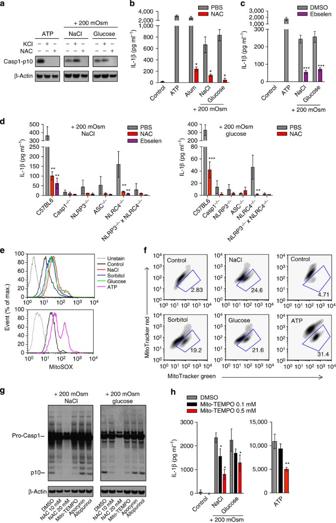Figure 5: Hyperosmotic stress activates inflammasomes via mitochondrial ROS. (a–d) LPS-primed BMDMs generated from wild-type (C57BL/6) mice only (a–c), or also from Casp1−/−, NLRP3−/−, ASC−/−NLRC4−/−or NLRP3−/−× NLRC4−/−mice (d) were incubated for 3 h (a) or overnight (b–d) in isotonic conditions (control) or hypertonic conditions (+200 mOsm) by adding NaCl, sorbitol or glucose, or stimulated with ATP (5 mM) for 30 min (a) or 2 h (b,c), or with alum (250 μg ml−1) for 4 h (b), in the presence of 100 mM extracellular KCl or after pretreatment with 10 mMN-acetyl-L-cysteine (NAC) or 50 μM ebselen. Cell lysates or media supernatants were analysed by immunoblotting for cleavage of caspase-1 (a; see alsoSupplementary Fig. 2b) or ELISA for IL-1β secretion (b–d), respectively. (e,f) Primed BMDMs incubated hypertonically or with ATP as inawere labelled with MitoSOX (which fluoresces upon oxidation by mitochondria-associated ROS) for mitochondrial ROS levels (e) or with MitoTracker Green (which stains the lipid membrane of the mitochondria) and MitoTracker Red (which fluoresces upon oxidation in respiring mitochondria) for dysfunctional mitochondria (f). Density plots (f) of fluorescence-activated cell sorting analysis show the percentages of dysfunctional mitochondria (MitoTracker Green+high, MitoTracker Red+low). (g,h) After pretreatment with NAC (10 or 20 mM), Mito-TEMPO (0.1 or 0.5 mM), apocynin (100 μM) or allopurinol (100 μM), primed macrophages were incubated hypertonically as inafor 3 h (g) or overnight (h), or stimulated with ATP (5 mM) for 2 h (h). Cleavage of caspase-1 (g) or IL-1β secretion (h) was assayed as inaorb, respectively. Data are representative of at least three independent experiments. Data indicate mean±s.d. of quadruplicates. Student’st-test: *P≤0.05, **P≤0.01, ***P≤0.001. Figure 5: Hyperosmotic stress activates inflammasomes via mitochondrial ROS. ( a – d ) LPS-primed BMDMs generated from wild-type (C57BL/6) mice only ( a – c ), or also from Casp1 −/− , NLRP3 −/− , ASC −/− NLRC4 −/− or NLRP3 −/− × NLRC4 −/− mice ( d ) were incubated for 3 h ( a ) or overnight ( b – d ) in isotonic conditions (control) or hypertonic conditions (+200 mOsm) by adding NaCl, sorbitol or glucose, or stimulated with ATP (5 mM) for 30 min ( a ) or 2 h ( b , c ), or with alum (250 μg ml −1 ) for 4 h ( b ), in the presence of 100 mM extracellular KCl or after pretreatment with 10 mM N -acetyl- L -cysteine (NAC) or 50 μM ebselen. Cell lysates or media supernatants were analysed by immunoblotting for cleavage of caspase-1 ( a ; see also Supplementary Fig. 2b ) or ELISA for IL-1β secretion ( b – d ), respectively. ( e , f ) Primed BMDMs incubated hypertonically or with ATP as in a were labelled with MitoSOX (which fluoresces upon oxidation by mitochondria-associated ROS) for mitochondrial ROS levels ( e ) or with MitoTracker Green (which stains the lipid membrane of the mitochondria) and MitoTracker Red (which fluoresces upon oxidation in respiring mitochondria) for dysfunctional mitochondria ( f ). Density plots ( f ) of fluorescence-activated cell sorting analysis show the percentages of dysfunctional mitochondria (MitoTracker Green +high , MitoTracker Red +low ). ( g , h ) After pretreatment with NAC (10 or 20 mM), Mito-TEMPO (0.1 or 0.5 mM), apocynin (100 μM) or allopurinol (100 μM), primed macrophages were incubated hypertonically as in a for 3 h ( g ) or overnight ( h ), or stimulated with ATP (5 mM) for 2 h ( h ). Cleavage of caspase-1 ( g ) or IL-1β secretion ( h ) was assayed as in a or b , respectively. Data are representative of at least three independent experiments. Data indicate mean±s.d. of quadruplicates. Student’s t -test: * P ≤0.05, ** P ≤0.01, *** P ≤0.001. 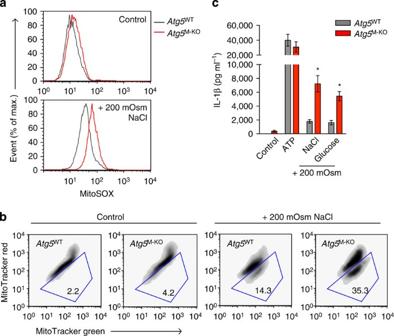Figure 6: Mitophagy controls hyperosmotic stress-induced inflammasome activation. (a–c) LPS-primed BMDMs generated from Atg5flox/flox(Atg5WT) or Atg5flox/floxLysM-Cre (Atg5M-KO) mice were incubated for 3 h (a,b) or overnight (c) in isotonic conditions (control) or hypertonic conditions (+200 mOsm) by adding NaCl or glucose, and labelled with MitoSOX (which fluoresces upon oxidation by mitochondria-associated ROS) for mitochondrial ROS levels (a) or MitoTracker Green (which stains the lipid membrane of the mitochondria) and MitoTracker Red (which fluoresces upon oxidation in respiring mitochondria) for dysfunctional mitochondria (b) or assayed for IL-1β in media supernatants by ELSIA (c). Density plots of fluorescence-activated cell sorting analysis show the percentages of dysfunctional mitochondria (MitoTracker Green+high, MitoTracker Red+low). Data are representative of two independent experiments. Data indicate mean±s.d. of quadruplicates. Student’st-test: *P≤0.05. Full size image Figure 6: Mitophagy controls hyperosmotic stress-induced inflammasome activation. ( a – c ) LPS-primed BMDMs generated from Atg5 flox/flox (Atg5 WT ) or Atg5 flox/flox LysM-Cre (Atg5 M-KO ) mice were incubated for 3 h ( a , b ) or overnight ( c ) in isotonic conditions (control) or hypertonic conditions (+200 mOsm) by adding NaCl or glucose, and labelled with MitoSOX (which fluoresces upon oxidation by mitochondria-associated ROS) for mitochondrial ROS levels ( a ) or MitoTracker Green (which stains the lipid membrane of the mitochondria) and MitoTracker Red (which fluoresces upon oxidation in respiring mitochondria) for dysfunctional mitochondria ( b ) or assayed for IL-1β in media supernatants by ELSIA ( c ). Density plots of fluorescence-activated cell sorting analysis show the percentages of dysfunctional mitochondria (MitoTracker Green +high , MitoTracker Red +low ). Data are representative of two independent experiments. Data indicate mean±s.d. of quadruplicates. Student’s t -test: * P ≤0.05. Full size image We next tested whether ROS is required for both NLRP3 and NLRC4 activation. As expected, in NLRC4-deficient BMDMs, ROS inhibitors significantly suppressed IL-1β secretion ( Fig. 5d ), confirming that NLRP3 activation by hyperosmotic stress is mediated via ROS. Intriguingly, BMDMs lacking NLRP3 were also sensitive to the inhibition by the ROS inhibitors ( Fig. 5d ), suggesting that, unlike the activation by cytosolic flagellin, which is ROS independent ( Supplementary Fig. 8 ), NLRC4 activation induced by hyperosmotic stress might also require ROS. Future study will need to address whether NLRP3 and NLRC4 are engaged into the same complex in response to ROS elevation for optimal induction of caspase-1 activation by hyperosmotic stress. Hyperosmotic stress has been shown to increase mitochondrial ROS production [32] . We therefore hypothesized that mitochondrial ROS contributes to the inflammasome activation by hyperosmotic stress. To examine ROS levels in the mitochondria upon hyperosmotic challenge, we used the mitochondria-specific ROS indicator MitoSOX to selectively detect superoxide in the mitochondria of live cells. MitoSOX is targeted to mitochondria and its oxidation by superoxide leads to the generation of red fluorescence. Our data showed that MitoSOX fluorescence was enhanced by hyperosmotic challenge in BMDMs ( Fig. 5e ), indicating that hyperosmotic stress induces mitochondrial ROS generation. To test if the increase in mitochondrial ROS was accounted for by accumulation of dysfunctional mitochondria, we then used two types of mitochondria-specific fluorescent labels to distinguish respiring (MitoTracker Red) versus total (MitoTracker Green) mitochondria. An increase in dysfunctional mitochondria (MitoTracker Green +high , MitoTracker Red +low ) was observed in BMDMs incubated in hypertonic conditions ( Fig. 5f ). This is in line with the loss of mitochondrial membrane potential observed by using tetramethylrhodamine methyl ester (TMRM) staining ( Supplementary Fig. 9 ). These data suggest that inflammasome activating ROS is generated by mitochondria. In support of this, caspase-1 activation by hyperosmotic stress was inhibited by the mitochondrial ROS inhibitor MitoTEMPO, but not by the nicotinamide adenine dinucleotide phosphate (NADPH) oxidase inhibitor apocynin or the xanthine oxidase inhibitor allopurinol ( Fig. 5g ). Hypertonic stress-induced caspase-1 activation was also normal in BMDMs lacking gp91-phox, the subunit of NADPH oxidase ( Supplementary Fig. 10 ). MitoTEMPO also inhibited IL-1β secretion ( Fig. 5h ). Combined with increased mitochondrial ROS production ( Fig. 5e ) and increase in dysfunctional (non-respirating) mitochondria ( Fig. 5f ), these data suggest that ROS produced from damaged mitochondria upon hyperosmotic stress is involved in inflammasome activation. Autophagy is one of the major pathways by which dysfunctional or damaged mitochondria are cleared from the cells through a process known as mitophagy [33] . Mitophagy has been shown to control the activation of NLRP3 inflammasome by several stimuli [34] , [35] , [36] . Consistent with these findings, Atg5-deficient BMDMs had increased mitochondrial ROS, accumulated dysfunctional mitochondria and enhanced IL-1β secretion in response to hypertonic stress, compared with wild-type BMDMs ( Fig. 6a–c ). These data suggest that mitophagy plays a role in regulation of the hyperosmotic stress-induced inflammasome activation. Collectively, the above findings have provided insights into the mechanism of inflammasome activation triggered by hyperosmotic stress. However, the upstream mechanism before inflammasome activation remained unclear. It is likely that the upstream mechanism leading to inflammasome activation couples with signalling pathways that act to sense hyperosmolarity in extracellular environments and are not macrophage-specific but common to many, if not all, cell types. We have considered various potential signalling pathways, which have been reported in different cell types previously by others, and tested a number of those. We evaluated their contribution to the inflammasome activation under hypertonic conditions by using inhibitors or BMDMs generated from knockout mice, that are specific for or lacking key signalling mediators or ion channels ( Supplementary Table 1 ). However, none of these inhibitions or gene deficiencies in macrophages prevented the activation of inflammasome trigger by hyperosmotic stress ( Supplementary Table 1 and Supplementary Figs 11–17 ), suggesting that the upstream mechanism leading to inflammasome activation is either redundant or mediated via an unknown pathway. Further research will be needed to clarify this aspect. Inflammasome activation promotes Th17 response in mice on high-salt diet High dietary salt (NaCl) intake has been associated with pathological conditions including enhanced inflammation in humans and mice. Recent studies in animals have shown that high-salt diets can lead to interstitial hypertonic salt accumulation in skin [37] , and promote tissue inflammation by enhancing Th17 cell differentiation in lymphoid tissues in mice with experimental autoimmune encephalomyelitis [38] , [39] . The Th17 differentiation was dependent on T-cell expression of the salt-induced serum glucocorticoid kinase 1 [38] , [39] . Given our findings that hypertonic stress promotes IL-1β production and the established role of IL-1β in Th17 differentiation [40] , we asked whether inflammasome-mediated salt-sensing mechanism in tissue compartments is involved in the induction of Th17 response in vivo . To address this, we examined whether caspase-1 is required for the Th17 polarization in mice maintained on high-salt diet. Consistent with the previous studies [38] , [39] , we observed enhanced Th17 response in high-salt diet mice immunized with ovalbumin (OVA)/LPS. Specifically, we detected increased Il17a but not Ifng mRNA expression and higher numbers of IL-17A-expressing CD4 + T cells in draining lymph nodes from wild-type mice fed high-salt diet as compared with controls ( Fig. 7a,b ). Furthermore, draining lymph node cells from wild-type mice on high-salt diet showed significantly enhanced IL-17A but not interferon-γ cytokine secretion upon OVA re-stimulation in vitro ( Fig. 7c and Supplementary Fig. 18 ), indicating enhanced in vivo induction of antigen-specific Th17 cells. Most importantly, these enhancements of Th17 response by high-salt diet were abolished in caspase-1-deficient mice ( Fig. 7a–c ), indicating that caspase-1 activation is required for the enhanced Th17 response. These data support the idea that inflammasome activation plays an important physiological role in sensing hypertonic salt accumulation in tissue compartments and promoting Th17 responses. 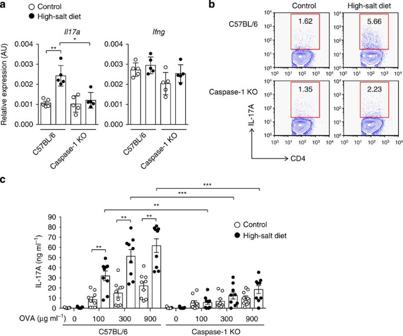Figure 7: Inflammasome activation promotes Th17 response in mice on high-salt diet. (a–c) Wild-type mice (C57BL/6) or caspase-1-deficient mice (Caspase-1 KO) fed high-salt or control diet (each group,n=9) were immunized with OVA/LPS for 7 days. Single-cell suspension prepared from draining lymph nodes was analysed forIl17aandIfngmRNA expression by quantitative reverse transcription–PCR (a) or intracellular IL-17A production in CD4+T cells by fluorescence-activated cell sorting (FACS) analysis (b), or re-stimulatedin vitrowith the indicated concentrations of OVA for 2 days and supernatants were analysed for IL-17A by ELISA (c). Data are mean±s.d. for pooled group of mice. Contour plots of FACS analysis show the percentages of IL-17-producing CD4+ T cells. Student’st-test: *P≤0.05, **P≤0.01, ***P≤0.001. Figure 7: Inflammasome activation promotes Th17 response in mice on high-salt diet. ( a – c ) Wild-type mice (C57BL/6) or caspase-1-deficient mice (Caspase-1 KO) fed high-salt or control diet (each group, n =9) were immunized with OVA/LPS for 7 days. Single-cell suspension prepared from draining lymph nodes was analysed for Il17a and Ifng mRNA expression by quantitative reverse transcription–PCR ( a ) or intracellular IL-17A production in CD4 + T cells by fluorescence-activated cell sorting (FACS) analysis ( b ), or re-stimulated in vitro with the indicated concentrations of OVA for 2 days and supernatants were analysed for IL-17A by ELISA ( c ). Data are mean±s.d. for pooled group of mice. Contour plots of FACS analysis show the percentages of IL-17-producing CD4+ T cells. Student’s t -test: * P ≤0.05, ** P ≤0.01, *** P ≤0.001. Full size image The identification of a family of cytosolic innate immune sensors NLRs has led to an explosion of interest in understanding the functional role of these innate immune signalling pathways [12] , [13] , [41] , [42] . The large number of known activators of NLRP3 inflammasome, either of biological or abiotic origin, makes it highly unlikely that the NLRP3 inflammasome directly senses the stimuli that can activate it. Instead, it is now generally acknowledged that NLRP3 activation occurs mainly as a consequence of a common form of cellular stress events elicited by these stimuli. This notion is supported by recent studies where an innate immune activation through NLRP3 inflammasome can be triggered in ER-stress and oxidative-stress conditions [43] , [44] . Collectively, these observations support the notion that NLRP3 inflammasomes may function to detect cellular and tissue stress conditions and convert them into inflammatory responses. These inflammatory responses normally operate to promote defence and adaptation to stress conditions, but in chronic settings can become detrimental giving rise to a variety of inflammatory pathologies. Here we provide evidence for a inflammasome-dependent innate immune response to hyperosmotic stress and suggest that both NLRP3 and NLRC4 act to sense hyperosmolality of tissue microenvironment and mediate inflammatory responses, including neutrophil recruitment, and adaptive Th17 responses. Our data implicating macrophages in sensing hyperosmotic stress and releasing mature IL-1β suggest that adaptation responses to physiologic hyperosmotic stress involve inflammatory components. It is in line with the observations from early studies, showing production of cytokines, including IL-1β in response to hyperosmotic stress in human peripheral blood mononuclear cells (PBMCs) and epithelial cells [45] , [46] . Here we show that this inflammatory response is triggered through the activation of caspase-1 by inflammasomes. Intriguingly, unlike the majority of known stimuli that activate the inflammasome through a specific NLR, hyperosmotic stress activates the inflammasome through both NLRP3 and NLRC4. Although the involvement of multiple NLRs has been previously reported [20] , [47] , [48] , it remains to be addressed how both NLRP3 and NLRC4 are engaged by a single stimulus via a pathway that involves ROS. One possibility is that NLRP3 and NLRC4 assemble into the same complex that is somehow involved in optimal induction of caspase-1 activation by hyperosmotic stress. Alternatively, there could be two distinct pathways activated by hyperosmotic stress, which are mediated via NLRP3 and NLRC4 separately and both dependent on ROS. Caspase-1 activation through the inflammasome formation was only observed in macrophages but not other cell types such as the fibroblast and epithelial cells tested in this study. It is likely due to the fact that NLRP3 and NLRC4 are specifically expressed in macrophages. This suggests that macrophages utilize this specific array of NLRs to sense environmental hyperosmolality and mediate inflammatory responses. Moreover, this macrophage-specific sensing pathway could be uncoupled from the typical cell-autonomous stress response pathway as caspase-1 activation in macrophages was not required for the adaptation to, and survival of osmotic stress ( Supplementary Fig. 4b ). Exposure of cells to hyperosmotic conditions causes numerous cellular stress events that could potentially activate the inflammasome formation, for example, cytoskeletal rearrangement due to cell shrinkage, solute influx (for example, ions, water) and ROS production. A recent study has demonstrated that, under hypo-osmotic conditions, NLRP3 inflammasome is activated through low intracellular K + (for example, K + efflux) that is controlled by transient receptor potential (TRP) channels such as TRP vanilloid 2 (TRPV2) [49] . Interestingly, here we show that inflammasome activation was affected neither by blocking K + efflux nor by using macrophages deficient in TRPV2. Instead, the activation was inhibited by NAC and MitoTEMPO, indicating that ROS generated by mitochondria is responsible for activating the inflammasome under the hyperosmotic stress conditions. Moreover, it is regulated by autophagy through maintaining mitochondrial homeostasis (that is, mitophagy) and thus suppressing mitochondrial ROS production. Together, these findings suggest that, although both hypo-osmotic and hyper-osmotic stresses cause cell volume perturbation (cell swelling and shrinkage, respectively), they activate inflammasome formation through different mechanisms, where macrophages have evolved to employ different strategies to sense cellular perturbations in order to activate caspase-1 through inflammasomes. The hyperosmotic stress response is critical not only to the survival of unicellular organisms, but it also has physiological functions in multicellular organisms, for example, in the kidney, where tubular epithelium is continuously exposed to extraordinarily high levels of osmolality (>1,000 mOsm) [1] . Cells in other tissues also deal with variations in osmolarity of their microenvironment, such as interstitial fluid. A previous study has shown that compartments in lymphoid tissues have higher osmolality relative to blood, which is maintained within tightly regulated range (for example, 285–295 mOsm in humans), and a failure in sensing hyperosmotic stress can lead to impaired adaptive immune responses [50] , indicating that lymphocytes-mediated immunity is contingent on adaptation to physiologic hyperosmotic stress. Also, the osmolality in tissue compartments can be affected by high dietary salt intake [37] . Thus, our data indicate that macrophage inflammasomes can sense hypertonic stress caused by high salt diet, promoting local inflammation and induction of Th17 response. Th17 response has been implicated in the pathogenesis of inflammation and autoimmunity in humans and mice [40] . Recent studies have shown that high salt diet promotes Th17 cell differentiation thereby contributing to the pathogenesis of autoimmune diseases [38] , [39] . T-cell expression of the salt-induced serum glucocorticoid kinase 1 has been shown to be important for this response [38] , [39] . Our study complements these reports by demonstrating innate sensing component for the hypertonic stress-induced Th17 response, which is likely mediated through the effect of IL-1β on Th17 cell differentiation. The findings reported here thus suggest inflammasomes and mitochondrial ROS as additional targets for Th17-mediated inflammatory diseases associated with high dietary salt intake. Mice Caspase-1-deficient ( Casp1 −/− ) mice, NLRP3-deficient ( Nlrp3 −/− ) mice, ASC-deficient ( Asc −/− ) mice and NLRC4-deficient ( Nlrc4 −/− ) mice were provided by Richard Flavell (Yale University, New Haven, CT, USA). NLRP3/NLRC4-double-deficient ( Nlrp3 −/− x Nlrc4 −/− ) mice were generated in our laboratory. Atg5 flox/flox mice were kindly provided by Dr Mizushima (Tokyo Medical and Dental University). Atg5 flox/flox LysM-Cre + mice were gifts of Herbert Virgin (Washington University, ST Louis, MO, USA). NKCC1-deficient ( Nkcc1 −/− ) mice, PIP5KIβ-deficient ( Pip5k1b −/− ) mice, PLCβ2/PLCβ3-double-deficient ( Plcb2 −/− x Plcb3 −/− ) mice and TRPV2-deficient ( Trpv2 −/−) mice were kindly provided by Gary Shull (University of Cincinnati), Charles Abrams (University of Pennsylvania, Philadelphia, PA, USA), Dan Wu (Yale University, New Haven, CT, USA), Michael Caterina (Johns Hopkins University, Beltimore, MD, USA), respectively. C57BL/6 mice, IL-1R-deficient ( Il1r1 −/− ) mice, gp91phox-deficient ( Cybb −/− ) mice and P2X 7 -deficient (P2x7 −/− ) mice were from the Jackson Laboratories. Mice doubly deficient in NLRP3 and NLRC4 were generated from Nlrp3 −/− mice and Nlrc4 −/− mice. All mice were bred and housed in accordance with National Institutes of Health- and Yale Animal Resources Center (YARC)-approved guidelines, and all studies involving mice were performed in accordance with approved Yale University Institutional Animal Care and Use Committee protocols and procedures. Reagents Allopurinol, apocynin, ATP, C. difficile Toxin B, E. coli LPS, EIPA, glucose, incomplete Freund’s adjuvant, NAC, sorbitol, OVA, ouabain and wortmanin were from Sigma-Aldrich. Alum (Imject alum adjuvant) was from Pierce. SB203580 and JNK Inhibitor II were from Calbiochem. Hoechst, MitoTracker Green, MitoTracker Red CMXRos, MitoSOX and TMRM were from Molecular Probes. MitoTEMPO was from Enzo Life Sciences. NaCl was from American Bioanalytical. Green-fluorescent FLICA was from Immunochemistry Technologies. Flow cytometry antibodies used include Ly-6G (clone RB6-8C5), F4/80 (clone BM8) and IL-17A (clone eBio17B7), all from eBioscience. Cells and cell treatments Bone marrow cells isolated from the above mice strains between 6 and 12 weeks of age were grown at 37 °C in a humidified incubator in RPMI-1640 medium containing 10% FCS and 30% L929 supernatant for 7–8 days. Differentiated bone marrow-derived macrophages (BMDMs) were re-plated into 24- or 96-well plates in RPMI-1640 medium containing 10% FCS and 20% L929 supernatant 16–20 h before cell treatments. To induce hyperosmotic stress, cells were switched to hypertonic conditions made by adding a non-permeant solute such as NaCl, sorbitol or glucose into the culture medium. For an increase of 0.2 milli-osmolality (that is,+200 mOsm kg −1 H 2 O), 100 mM NaCl, 200 mM sorbitol or 200 mM glucose was added. Cells maintained in the regular culture medium (that is, ∼ 300 mOsm kg −1 H 2 O) were used as controls for isotonic conditions. In some experiments, LPS-primed macrophages were incubated in the presence of KCl (100 mM), or pretreated for 30 min with NAC (10 or 20 mM), ebselen (50 μM), MitoTEMPO (0.1 or 0.5 μM), apocynin (100 μM) or allopurinol (100 μM) before the stress induction. Cell volume Cell volume measurements were performed by using a Coulter Counter Model Z2 (Beckman). Cells in suspension were diluted in PBS (isotonic control) or PBS with 100 mM NaCl, 200 mM sorbitol or 200 mM glucose (hypertonic conditions;+200 mOsm kg −1 H 2 O) and incubated for the indicated times. Cells were analysed according to the manufacturer’s instructions. Cell sizes were also observed by differential interference contrast microscopy. Microarray analysis BMDMs were incubated in hypertonic conditions by adding 100 mM NaCl, or 200 mM sorbitol, or stimulated with 100 ng ml −1 LPS for 3 h and harvested into Trizol Reagent (Invitrogen). Sample preparation and hybridization to Illumina MouseWG-6 Expression BeadChip were performed at the Yale W. M. Keck facility. Gene expression heat map was created by using Cluster 3.0 and Java TreeView softwares. Cytokine production BMDMs were primed with or without LPS for 3 h and incubated in hypertonic conditions as described above. Supernatants were harvested after overnight incubation. Release of proinflammatory cytokines was measured by ELISA using capture and detection antibodies against IL-6, IL-1α (BD Pharmingen), or IL-1β (eBioscience), according to the manufacturer’s protocol. LPS-primed BMDMs stimulated with ATP (5 mM) or Alum (250 μg ml −1 ) for 2 or 6 h, respectively, were used as positive controls for IL-1β secretion. In vivo peritonitis Age- and sex-matched mice of the indicated mouse strains between 6 and 8 weeks of age were injected i.p. with 0.15 or 0.35 M NaCl solution at 0.4 ml per 10 g of body weight. After 16 h, peritoneal lavage cells were stained with fluorescently conjugated monoclonal antibodies against Ly-6G (clone RB6-8C5) and F4/80 (clone BM8; eBioscience), and analysed by flow cytometry as described above. The absolute number of neutrophils (Ly-6G-positive, F4/80-negative) was determined by using CountBright counting beads (Molecular Probes) according to the manufacturer’s protocol. Western blotting Electrophoresis of proteins was performed using NuPAGE system (Invitrogen) according to the manufacturer’s protocol. Briefly, BMDMs primed with LPS for 3 h were incubated in hypertonic conditions as described above for 3 h, lysed in lysis buffer (20 mM HEPES, 150 mM NaCl, 10% glycerol, 1% Triton X-100 and 1 mM EDTA, and 1 × protease inhibitor cocktails (Roche)) and stored at −20 °C until analysed. For caspase-1 release, media supernatants were harvested after overnight incubation in hypertonic conditions as described above and stored at −20 °C until analysed. Before electrophoresis, whole-cell lysates or media supernatants were diluted with 5 × protein sample buffer (125 mM Tris-HCl (pH 6.8), 10% SDS, 50% glycerol, 0.06% bromophenol blue and 1% β-mercaptoethanol) and incubated at 72 °C for 10 min. Proteins were separated on 4–12% NuPAGE gels and transferred to polyvinylidene difluoride membrane (Millipore). To detect caspase-1, a rabbit polyclonal anti-mouse caspase-1 p10 antibody (sc-514; Santa Cruz Biotechnology) was used. LPS-primed BMDMs stimulated with ATP (5 mM) or Alum (250 μg ml −1 ) for 30 min or 4 h, respectively, for caspase-1 activation in whole-cell lysates, or for 2 or 6 h, respectively, for caspase-1 release in media supernatants were used as positive controls. Flow cytometry MitoSOX, MitoTracker Green, MitoTracker Red CMXRos and TMRM staining were performed according to the manufacturer’s instructions (Invitrogen). Data were acquired with a FACSCalibur flow cytometer (BD Biosciences) and analysed with FlowJo software (Tree Star). High-salt diet and immunizations Age- and sex-matched mice of the indicated mouse strains between 6 and 8 weeks of age were fed normal chow (Harlem Laboratories; TD. 96208 laboratory diet) and tap water ad libitum (control group) or sodium-rich chow (Harlem Laboratories; TD. 92034 laboratory diet) and tap water containing 1% NaCl ad libitum (high-salt group) for 4 weeks, and immunized subcutaneously in the rear footpads with 5 μg LPS and 50 μg OVA emulsified in incomplete Freund’s adjuvant. Popliteal lymph nodes were isolated from mice after 6 days later, and single-cell suspensions were made by grinding the lymph nodes between two sterile frosted slides and filtered through 70-μm cell strainer. Real-time PCR Total RNA was isolated from single-cell suspensions using RNeasy kit (Qiagen). Poly(A)-tailed mRNA was reverse transcribed using SMART MMLV reverse transcriptase (Clontech). PCR was performed using intron-spanning gene-specific primers and SYBR green master mix (Quanta) on Bio-Rad real-time PCR machine. The expression levels of target genes were normalized to Gapdh . Sequences of the primers used in this study are shown in the Supplementary Table 2 . Statistical analysis Plotting of data and statistical analysis were performed using Graphpad Prism 4.0 software, and statistical significance was determined by unpaired two-tailed Student’s t -test, where P <0.05 was considered statistically significant. How to cite this article: Ip, W. K. E. et al . Macrophages monitor tissue osmolarity and induce inflammatory response through NLRP3 and NLRC4 inflammasome activation. Nat. Commun. 6:6931 doi: 10.1038/ncomms7931 (2015).